Strain-controlled magnetic domain wall propagation in hybrid piezoelectric/ferromagnetic structures The control of magnetic order in nanoscale devices underpins many proposals for integrating spintronics concepts into conventional electronics. A key challenge lies in finding an energy-efficient means of control, as power dissipation remains an important factor limiting future miniaturization of integrated circuits. One promising approach involves magnetoelectric coupling in magnetostrictive/piezoelectric systems, where induced strains can bear directly on the magnetic anisotropy. While such processes have been demonstrated in several multiferroic heterostructures, the incorporation of such complex materials into practical geometries has been lacking. Here we demonstrate the possibility of generating sizeable anisotropy changes, through induced strains driven by applied electric fields, in hybrid piezoelectric/spin-valve nanowires. By combining magneto-optical Kerr effect and magnetoresistance measurements, we show that domain wall propagation fields can be doubled under locally applied strains. These results highlight the prospect of constructing low-power domain wall gates for magnetic logic devices. The prospect of controlling local magnetization using electric fields for ultra-low-power spintronics has resulted in a new research direction that involves multiferroic and magnetoelectric materials [1] , [2] , [3] , [4] , [5] , [6] . However, existing approaches involving natural multiferroics are either limited by weak ferromagnetism at room temperature [7] or are effective only at low temperatures [8] , [9] . One promising avenue to circumvent such issues concerns the use of strain-mediated coupling in piezoelectric/magnetostrictive bilayer structures [10] , [11] , [12] , [13] , [14] , [15] , [16] . In such structures, the applied voltage across the film thickness generates a uniaxial strain in the piezoelectric layer that is transferred to the magnetostrictive nanomagnet, resulting in a change in its magnetic properties. It has been shown theoretically that this can form the basis of ultra-low-power computing and signal processing towards possible applications for energy harvesting [17] , [18] . In this context, first investigations of individual switching events under applied voltages have been reported in thin-film FeGa/BaTiO 3 bilayer structures [19] . However, the difficulty to integrate such complex heterostructures into electrically controlled nanoscale devices has precluded the demonstration of local manipulation of single nanomagnet that would be an essential step towards the magnetoelectric control of spintronic devices. A promising approach towards high-density magnetic memories [20] , [21] and spin logic elements [22] involves the propagation of domain walls (DWs) in magnetic nanowires. In this work, we demonstrate that DW motion can be electrically controlled at room temperature using strain-mediated magnetoelectric coupling in piezoelectric/ferromagnetic nanostructures. We first describe a device geometry that allows for an efficient transfer of a strong local strain to the ferromagnetic stripe. By using conventional three-dimensional ferromagnetic spin valves (SVs), in conjunction with the commonly used piezoelectric material PbZr 0.5 Ti 0.5 O 3 (PZT), we show that the energy barrier for DW motion can be doubled under reasonable applied electric fields. We show how such functionality can be exploited in a DW gate, which could serve to generate Boolean logic functions or stabilize DWs in memory applications. Hybrid PZT/ferromagnetic device structure and transport measurements A straightforward means of obtaining high magnetoelectric coupling involves encapsulating the magnetic nanodevice inside a piezoelectric environment [23] . However, two important hurdles must be overcome to achieve this goal. First, ceramic piezoelectric layers, like PZT, require high temperature deposition or post annealing (>400 °C) under severe oxidation conditions [24] , which inevitably degrade the magnetic properties. Second, the clamping effect from the substrate limits the crystal stress in any solid-state device. In order to avoid these issues, we have focused on an approach based on the lateral geometry seen in Fig. 1 , which allows for memory and logic functions to be constructed using magnetic DWs in nanowires (see Supplementary Discussion . The sides of the piezoelectric bar are free to move but its bottom surface is clamped by the substrate, which does not allow for any global longitudinal compression. By applying a voltage, the electrical polarization rotates away from the growth direction [25] , which induces a strain ε xx >0 corresponding to an elongation in the bar width, particularly near the top surface where the magnetic wire is located. In addition, this geometry leads to a large accumulated strain ε yy at both longitudinal ends of electrodes. The induced strains along the x and y directions result in a local pinning potential for a DW, irrespective of the sign of the magnetostriction. 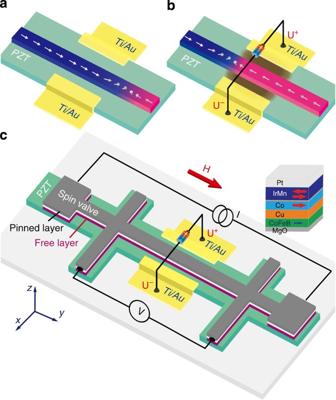Figure 1: Lateral approach used to manipulate magnetic domain wall through magnetoelectric coupling. (a) In the absence of applied voltages on the piezoelectric layer, the domain wall (DW) propagates freely in the magnetic stripe. (b) DW propagation in magnetic stripe can be controlled by voltages through lateral magnetoelectric coupling device. By applying a voltage onto the piezoelectric layer, a local stress is induced, followed by DW blockade. (c) Measurement configuration with hybrid PZT and spin-valve (SV) hall bar-shaped device, a single DW is injected from a large reservoir. The position of the DW is monitored by measuring the GMR between two electrodes. By applying a voltage on PZT, an induced stress results in a local modification of the domain wall dynamics. The SV multilayer structure is shown on the right. Figure 1: Lateral approach used to manipulate magnetic domain wall through magnetoelectric coupling. ( a ) In the absence of applied voltages on the piezoelectric layer, the domain wall (DW) propagates freely in the magnetic stripe. ( b ) DW propagation in magnetic stripe can be controlled by voltages through lateral magnetoelectric coupling device. By applying a voltage onto the piezoelectric layer, a local stress is induced, followed by DW blockade. ( c ) Measurement configuration with hybrid PZT and spin-valve (SV) hall bar-shaped device, a single DW is injected from a large reservoir. The position of the DW is monitored by measuring the GMR between two electrodes. By applying a voltage on PZT, an induced stress results in a local modification of the domain wall dynamics. The SV multilayer structure is shown on the right. Full size image In addition to the strain being transferred to the ferromagnetic nanowire, it is a desirable for magnetization reversal to be detected using a transport-based method, such as giant magnetoresistance (GMR), which would allow for such a device to be integrated into micro- and nanoelectronic components [26] . For this purpose, we used magnetic wires based on in-plane magnetized spin valves with composition free layer (FL)/Cu/Co, where two different FL materials were studied: a 5-nm-thick CoFeB layer and a 10-nm-thick composite permalloy/CoFeB layer. For a given lateral wire width of 700 nm, the different aspect ratio of the two systems gives rise to two distinct DW types: an asymmetric transverse DW configuration for the CoFeB system and a vortex wall for the permalloy/CoFeB system. The complete device structure is shown in Fig. 2a . 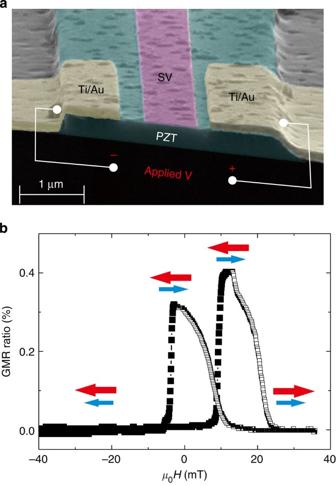Figure 2: Fabricated device structure and magnetic transport property of SV stripe. (a) Cross section of the device measured by scanning electron microscopy. SV stripe is located in the middle of PZT, and side electrodes are in a good contact with PZT side walls. (b) GMR loops of SV stripe, which is measured by sweeping an external magnetic fieldHalong easy axis. The free-layer and pinned-layer magnetization reversal with applied field are shown with solid black squares and open black squares, respectively. Figure 2: Fabricated device structure and magnetic transport property of SV stripe. ( a ) Cross section of the device measured by scanning electron microscopy. SV stripe is located in the middle of PZT, and side electrodes are in a good contact with PZT side walls. ( b ) GMR loops of SV stripe, which is measured by sweeping an external magnetic field H along easy axis. The free-layer and pinned-layer magnetization reversal with applied field are shown with solid black squares and open black squares, respectively. Full size image Transport measurements were first performed on the devices without any applied voltage, as shown in Fig. 2b . The typical GMR ratio is about 0.4% in the set of samples with 5 nm CoFeB as free layer, which is sufficiently high to detect DW motion with good precision in the free layer. The presence of an asymmetric high resistance state results from the pinned-layer (PL) magnetization that starts to reverse before the FL magnetization is fully reversed. The magnetization reversal of the PL is shifted to positive fields, owing to the presence of an exchange bias field μ 0 H ex =15 mT resulting from a coupling with the antiferromagnetic IrMn layer. For the FL, a slight shift towards positive fields (around 0.6 mT) can also be observed, which originates from an interlayer coupling between the two ferromagnetic layers [27] . The angular dependence of the coercive field of the free layer is consistent with the propagation of a single DW in the nanowire after being injected from a reservoir (see Supplementary Fig. S1 ). The hysteresis loop branch that corresponds to the reversal of the free layer can be then explained as follows: (1) injection of the DW at the first GMR electrode at H N , (2) propagation towards the PZT bars (bottom part of the branch), (3) propagation along the PZT bars (centre part of the branch) and then (4) propagation towards the second GMR electrode. Thus the coercive field here corresponds to the average propagation field along the PZT bar, which is about 6 mT at zero voltage. It is important to note that sharp steps in the GMR signal, which are typically associated with domain wall pinning and depinning, are not present in our samples for a number of reasons. First, there are potential contributions to the magnetoresistance from the Hall crosses. These structures consist of additional arms perpendicular to the wire in which wall propagation takes place. As a result, the MR curves contain an irreversible (sharp) component owing to wall propagation and a reversible (coherent rotation) part owing to magnetization rotation in the arms. Second, magnetization processes in the PL also contribute to the overall magnetoresistance signal. While the FL and PL loops are well separated in the full spin-valve films before patterning (as determined from magneto-optical Kerr effect measurements), the separation becomes less pronounced in the wire structures after patterning. As a result, the measured magnetoresistance signal contains both FL and PL reversal processes. Magneto-optical Kerr effect measurements of DW propagation In order to provide further evidence of DW propagation in our system, we performed spatially resolved magneto-optical Kerr effect (MOKE) measurements to study magnetization reversal at different regions along the magnetic wire. The experiments were conducted on samples with a 10-nm-thick permalloy/CoFeB free layer. The spatial resolution of the focused beams used is ~2 μm, which is sufficient to detect magnetization reversal inside and outside of the strained regions associated with the PZT electrodes. The experimental results are shown in Fig. 3 . We note that MOKE measurements for the patterned wires always show sharp hysteresis loops for the free layer, which is a key signature of magnetization reversal by DW propagation. When the spot is focused on the wire under unstrained PZT area ( Fig. 3a ), the coercive field is measured to be 7.5 mT. In contrast, the same measurement for a spot focused in the region in between the electrodes gives a coercive field of 11 mT, as shown in Fig. 3b . The coercive fields under strained PZT area are always larger than those under non-strained PZT area. The origin for a larger coercive field within the strained PZT region is unclear at this stage. We suspect that the coupling between the ferroelectric domains and the ferromagnetic domains may result in such an increase. The domain structure of the PZT areas covered by the gold electrode is also expected to be different from the uncovered areas. Furthermore, when the laser beam is focused in the unstrained area, the measured coercive fields show almost no variation with the applied voltage (see Supplementary Fig. S2b , the red stars). 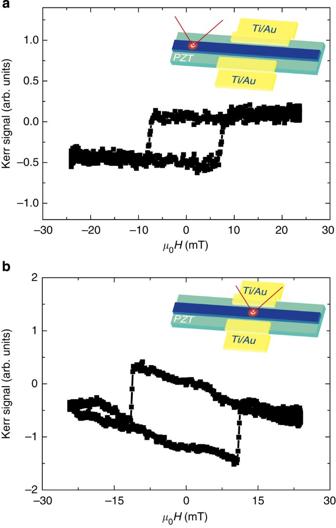Figure 3: Magneto-optical Kerr effect measurements of domain wall propagation. (a) Hysteresis loop determined from a spatially resolved MOKE measurement when the spot falls in a region outside of the PZT electrodes, which indicates a coercive field of 7.5 mT. (b) Hysteresis loop determined from a spatially resolved MOKE measurement when the spot falls in a region in between of the PZT electrodes, which indicates a coercive field of 11 mT. Insets: illustration of the position of the laser spot used in the spatially resolved MOKE measurement. Figure 3: Magneto-optical Kerr effect measurements of domain wall propagation. ( a ) Hysteresis loop determined from a spatially resolved MOKE measurement when the spot falls in a region outside of the PZT electrodes, which indicates a coercive field of 7.5 mT. ( b ) Hysteresis loop determined from a spatially resolved MOKE measurement when the spot falls in a region in between of the PZT electrodes, which indicates a coercive field of 11 mT. Insets: illustration of the position of the laser spot used in the spatially resolved MOKE measurement. Full size image From these data, we can confirm with a greater degree of certainty that domain nucleation occurs within the non-strained PZT area, as the coercive field is lower. Furthermore, the sharpness of the hysteresis loops indicates that magnetization reversal occurs through DW propagation. This lends further support to the physical picture we present here, that is, the magnetization reversal is initiated by domain nucleation and proceeds by DW propagation along the wire. However, MOKE measurements for our system in the strained area prove to be unreliable for studying DW propagation under applied voltages in detail for the following reasons. First, ferroelectric materials, like PZT, normally exhibit a hysteretic change of the birefringence with applied electric field based on their value of the remanent polarization [28] . The MOKE measurement of the strained PZT area under applied voltage contains a large background from the ferroelectric signal, which is not trivial to correct for. Second, the reflection of the laser beam from the two gold electrodes gives rise to an important source of additional noise. Third, the STO substrate used is transparent at a thickness of 1 mm, which means that the Faraday effect in the STO layer also contributes to total signal of the MOKE. As the longitudinal MOKE signal from the buried free layer of the nanowire is small, the MOKE measurements can only give qualitative information about changes in the coercive field H c under applied voltages. Given these difficulties, we choose to rely on magnetoresistance measurements to characterize DW propagation under applied voltages in our samples. Influence of induced strain on DW propagation The influence of the gate voltages on the DW propagation is illustrated in Fig. 4a . The initial state consists of an in-plane depolarized state of the PZT bar. The GMR ratio change with applied voltage is due to the PL magnetization reversal that occurs before the FL magnetization is fully reversed. The striking feature seen in Fig. 4a is a large increase of the coercivity of the free layer under stress. Following the magnetization reversal with magnetic field under voltage (see Supplementary Fig. S2a ), we observe first a change of slope of the ascending branch, showing a modification of the dynamics of DW motion only along the PZT bars. Note also that H N is not modified under voltage (see Supplementary Fig. S2b , black squares, which is consistent with MOKE measurements, red stars in Supplementary Fig. S2b ), which is consistent with the injection of the DW outside of the strained PZT area. The average propagation field H p as a function of applied voltage from –50 to 50 V (100 kV cm −1 ) was extracted at 50% of the total GMR ( Fig. 4b ). 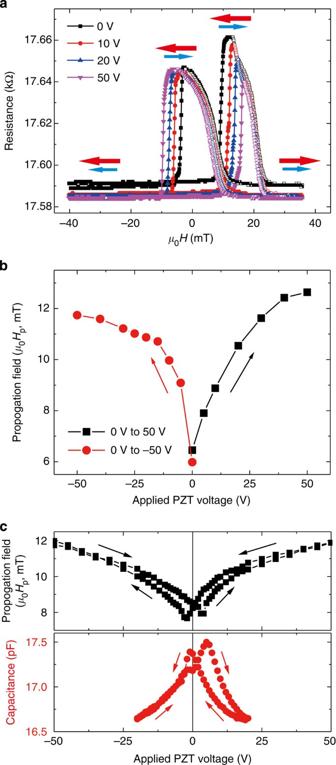Figure 4: GMR measurements of domain wall propagation in the free layer of 5 nm CoFeB. (a) Giant magnetoresistance loops with different applied voltages, which starts from a depolarized state of the PZT layer. (b) Propagation field in the free layer as a function of the voltage applied on the PZT layer. (c) Propagation field of free layer as measured by scanning the voltage applied on the PZT layer starting from −50 V (top panel) and C−V measurement of the PZT layer, starting from −20 V (bottom panel). Note that the propagation field of the FL doubles for an applied voltage of V PZT =±50 V. Figure 4: GMR measurements of domain wall propagation in the free layer of 5 nm CoFeB. ( a ) Giant magnetoresistance loops with different applied voltages, which starts from a depolarized state of the PZT layer. ( b ) Propagation field in the free layer as a function of the voltage applied on the PZT layer. ( c ) Propagation field of free layer as measured by scanning the voltage applied on the PZT layer starting from −50 V (top panel) and C−V measurement of the PZT layer, starting from −20 V (bottom panel). Full size image To further confirm that the change of H p is owing to the inverse magnetostrictive effect, the propagation field was directly compared with the capacitance of PZT under applied voltages. The H p was determined by scanning the voltage applied on the PZT layer as shown in the top panel of Fig. 4c . We clearly observe a butterfly shape as expected for a ferroelectric-related effect. The propagation field at 0 V is higher than in Fig. 4b , which is an indication of a remnant in-plane polarization of the PZT layer. C–V measurements of the PZT layer were performed at 1 MHz, as seen in the bottom panel of Fig. 4c . A butterfly shape is also clearly evidenced with a typical coercivity E c of about 3 V (6 kV cm −1 ). The observed asymmetrical switching is presumably linked to the asymmetric interface side contact generated from fabrication. We observe also that the hysteretic change of H p with voltage is linked to the switching of the two polarizations of the PZT layer, which is a clear indication of magnetoelectric coupling in our hybrid piezoelectric/ferromagnetic nanodevice. Note that any Joule heating can be excluded as the leakage current through the PZT layer is in the range of nA, H p increases with voltage and no increase in the spin-valve resistance is seen with applied voltages. These measurements were repeated for the 10-nm-thick permalloy/CoFeB FL system, in which a different DW structure is expected. Furthermore, the GMR ratio of 1.4% for this system is greater than the ratio for the 5-nm-thick CoFeB system, which allows for greater sensitivity for localizing the DW along the wire. The hysteresis curves obtained from magnetoresistance measurements are presented in Fig. 5 . In contrast to the first system, we observe clear plateaus in the FL switching under different applied voltages, while no plateaus are seen in the absence of applied voltages. The plateaus occur at positions representing 15–20% of the total MR variation, and are more obvious at higher voltages with larger strain, while independent of the sign of the applied voltage. These levels are consistent with DW pinning at the edges of the PZT electrodes, which is expected from electrical and micromagnetic modelling (see Supplementary Fig. S3 and Supplementary Discussion . The observation of plateaus in this particular system may be owing to two reasons. First, the permalloy/CoFeB FL system exhibits larger GMR value (that is, 1.4%, as opposed to 0.3% for the pure CoFeB FL system). Second, the vortex wall present is expected to be more sensitive to local pinning sites, owing to the compact nature of the wall structure. As such, it follows that the vortex wall will be more greatly affected by changes in these pinning sites owing to the applied strains. In Fig. 5c , one can observe that the change in the coercive field with applied voltage is less significant in comparison with the pure CoFeB system, as magnetostrictive effects are smaller in permalloy. Spatially resolved magneto-optical Kerr measurements confirm that magnetization reversal occurs by DW propagation through the strained PZT area in these samples (see Fig. 3 ). 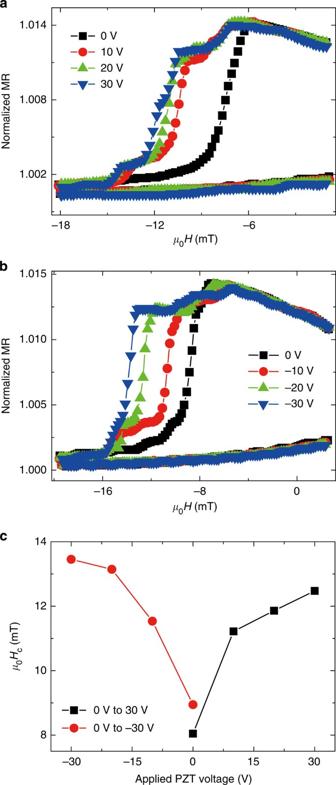Figure 5: GMR measurements of domain wall propagation in the free layer of 10 nm permalloy/CoFeB. (a) Zoom of giant magnetoresistance (GMR) loops with different applied voltages, which starts from a depolarized state of the PZT layer to 30 V, two clear plateaus are observed. (b) Zoom of GMR loops with different applied voltages, which starts from 0 to −30 V, two clear plateaus are also observed. (c) Propagation field in the free layer as a function of the voltage applied on the PZT layer. Figure 5: GMR measurements of domain wall propagation in the free layer of 10 nm permalloy/CoFeB. ( a ) Zoom of giant magnetoresistance (GMR) loops with different applied voltages, which starts from a depolarized state of the PZT layer to 30 V, two clear plateaus are observed. ( b ) Zoom of GMR loops with different applied voltages, which starts from 0 to −30 V, two clear plateaus are also observed. ( c ) Propagation field in the free layer as a function of the voltage applied on the PZT layer. Full size image We propose that our structure, which functions like a magnetic DW gate, can form the building block for generating Boolean logic functions. An example for a NOR gate is given in Fig. 6a . The principle is very similar to the concept of the magnetic shift register based on moving DWs in a racetrack geometry with spin-polarized currents [20] , [21] . The elementary logic device consists of a DW nanowire on top of a PZT bar, with a writing line to nucleate DWs, an electrical control ‘A’ for injecting spin-polarized currents into the wire, two inputs ‘B 0 ’ and ‘B 1 ’ that involve applied electric fields to the PZT layer and an output ‘C’ that involves detecting the local magnetization with a magnetic tunnel junction (MTJ). We point out that this system can be easily reconfigured to supply a logical NAND operation by simply starting the output ‘C’ in a ‘1’ initial state with an antiparallel magnetization configuration in the MTJ. As the two inputs ‘B 0 ’ and ‘B 1 ’ are identical, it is possible to construct as many of these as desired to obtain a multi-input (for example, eight bits) logic device. 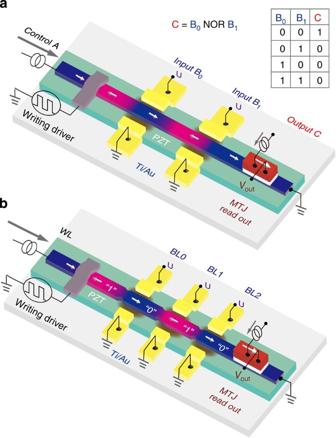Figure 6: Proposal of domain wall logic and domain wall memory. (a) Design of a multi-input NOR logic function by using voltage control of elementary DW gates. Control A is used for current-driven DW motion, and the writing line is used to generate a domain wall. Inputs B0and B1are piezoelectric-controlled DW gates, and output C serves as read out for the magnetization direction in the wire through the tunnelling magnetoresistance effect. The device functions as follows. First, a domain wall is nucleated in the wire with the Oersted field generated by the current flowing through the write line, with the output ‘C’ set to the low resistance state ‘0’ (parallel magnetization state of the MTJ). If either or both of the gate voltages ‘B0’ and ‘B1’ are applied (that is, in the ‘1’ state), then the induced anisotropy change at the gates concerned lead to a local pinning of the domain wall, which leaves the output ‘C’ in the ‘0’ state. However, if both gate voltages are off (inputs ‘B0’ and ‘B1’ set to ‘0’), then the generated domain wall can propagate free along the wire, driven by the spin-polarized currents controlled by ‘A’, leading to magnetization reversal at the output ‘C’ and thereby switching this state to ‘1’. This scheme corresponds to a logical NOR operation and NOR table is shown on top. (b) Design of a racetrack memory using voltage control of a DW gate. Proposed device scheme in which individual PZT electrodes supplement pinning sites defined by artificial notches. These electrodes act as bit lines (BL), as they allow individual domain walls to be pinned on demand by applied voltages, thereby allowing a content-addressable function to conventional racetrack memories. For example, in order to write the current state ‘1 0 1 0’ to final state ‘1 0 0 0’, the voltages on BL0 and BL2 are on and voltage on BL1 is off, by sending the domain wall-driven current (control A), the final state can be achieved. Figure 6: Proposal of domain wall logic and domain wall memory. ( a ) Design of a multi-input NOR logic function by using voltage control of elementary DW gates. Control A is used for current-driven DW motion, and the writing line is used to generate a domain wall. Inputs B 0 and B 1 are piezoelectric-controlled DW gates, and output C serves as read out for the magnetization direction in the wire through the tunnelling magnetoresistance effect. The device functions as follows. First, a domain wall is nucleated in the wire with the Oersted field generated by the current flowing through the write line, with the output ‘C’ set to the low resistance state ‘0’ (parallel magnetization state of the MTJ). If either or both of the gate voltages ‘B 0 ’ and ‘B 1 ’ are applied (that is, in the ‘1’ state), then the induced anisotropy change at the gates concerned lead to a local pinning of the domain wall, which leaves the output ‘C’ in the ‘0’ state. However, if both gate voltages are off (inputs ‘B 0 ’ and ‘B 1 ’ set to ‘0’), then the generated domain wall can propagate free along the wire, driven by the spin-polarized currents controlled by ‘A’, leading to magnetization reversal at the output ‘C’ and thereby switching this state to ‘1’. This scheme corresponds to a logical NOR operation and NOR table is shown on top. ( b ) Design of a racetrack memory using voltage control of a DW gate. Proposed device scheme in which individual PZT electrodes supplement pinning sites defined by artificial notches. These electrodes act as bit lines (BL), as they allow individual domain walls to be pinned on demand by applied voltages, thereby allowing a content-addressable function to conventional racetrack memories. For example, in order to write the current state ‘1 0 1 0’ to final state ‘1 0 0 0’, the voltages on BL0 and BL2 are on and voltage on BL1 is off, by sending the domain wall-driven current (control A), the final state can be achieved. Full size image The scheme described above could provide additional functionality to the racetrack memory device [20] , [21] , as shown in Fig. 6b . For the racetrack device, artificial constrictions are required to stabilize DWs against thermal fluctuations, but further downscaling of such geometries represents a technological challenge. Furthermore, high current densities are required to induce DW motion because of the strong pinning as a result of these constrictions. A possible solution to these issues could involve using voltage-induced strains to assist DW pinning at each of the constrictions in a racetrack device. When DW shifting is required, the voltages at all constrictions concerned can be set to zero, thereby leading to a reduced propagation field and therefore the requirement for lower current densities. The inclusion of the PZT electrodes would also endow the additional function of addressable content, as DWs in parts of the racetrack could be ‘clamped’ by applied electric fields, while walls in other parts could continue to be shifted along the wire. In the conventional racetrack memory, the storage is programmed strip-by-strip or word-by-word. This represents a serious drawback in comparison with random access memory in which each bit or storage element can be addressed individually. By combining with the read heads implemented on each individual information bit [29] , such a scheme could allow for each data in the magnetic stripe to be accessed for write and read operations, as in traditional random access memory [30] , where the PZT electrodes and magnetic nanowires are addressed, respectively, by bit lines and word lines. This additional functionality overcomes one of the key limitations of the conventional racetrack design, where DWs are driven in unison under applied currents without the storage being addressable individually [20] . Fabrication The devices consist of a PZT film with a lateral spin valve grown on top, and they were fabricated on vicinal SrTiO 3 (001) single-crystal substrates. The 400 nm PZT was first grown by pulsed laser deposition at 580 °C under 120 mTorr O 2 atmosphere [31] , [32] , [33] . It was then patterned into a 5-μm-wide Hall bar by optical lithography and ion milling using Ar and O 2 . The 700-nm-wide spin-valve stripe and the side gate electrodes in the middle part of the bar are fabricated by two steps of electron beam lithography and a subsequent lift-off process. The spin valves consisting 2(nm) MgO/FL/4 Cu/4 Co/0.3 Cu/8 IrMn/4 Pt, where the free layer (FL) is either 5 Co 40 Fe 40 B 20 or 5 permalloy/5 Co 40 Fe 40 B 20 , were grown by magnetron sputtering at 5.8 × 10 −4 mbar Ar under an in-plane bias field of 100 mT. The width of 700 nm for the spin-valve stripe was chosen to promote easy DW propagation by minimizing pinning owing to rough edges. For the spin-valve structure, a 2 nm MgO buffer was used to reduce the electrical field screening effect and domain coupling between the ferroelectric and ferromagnetic layers. A 0.3 nm layer of Cu was inserted between Co and IrMn to enhance the magnetic coupling [34] . The side gate electrodes (5 nm Ti/150 nm Au) were grown by e-beam evaporation and patterned to 4 μm (w) × 400 μm (l). Finally, contact electrodes with 10 nm Ti/300 nm Au were deposited using a lift-off process after optical lithography. Transport measurements An a.c. (10 μA) lock-in technique was used to obtain the GMR signal at room temperature under an applied voltage on the PZT. The hysteresis loops of GMR were measured by sweeping the magnetic field at a rate of 4 mT min −1 . Owing to the nature of ferroelectric domain structure, the voltages on PZT were applied in two ways. The first concerns the initial polarizing scan, which involves ramping the voltage from 0 V with an in-plane depolarized state to polarized states at high voltages (50 or –50 V). The second concerns the loop scan, which involves sweeping the voltage from an in-plane polarized state (−50 V) to 50 V and back to −50 V. The leakage currents measured during the voltage scans were measured to be in the nA range. Spatially resolved magneto-optical Kerr effect measurements A 2 μm-diameter-focused laser spot (thermally stabilized solid-state laser source at 660 nm with a power of about 100 mW) was placed on the spin-valve nanowire with an incidence angle of 45° in longitudinal MOKE geometry. The sinusoidal in-plane magnetic field along the nanowire is generated by a quadrupole electromagnet at a frequency of 3 Hz and an amplitude of 25 mT. How to cite this article: Lei, N. et al. Strain-controlled magnetic domain wall propagation in hybrid piezoelectric/ferromagnetic structures. Nat. Commun. 4:1378 doi: 10.1038/ncomms2386 (2013).